General rules for the arrangements and gating motions of pore-lining helices in homomeric ion channels The pore-lining helix (PLH) bundles are central to the function of all ion channels, as their conformational rearrangements dictate channel gating. Here we explore all plausible oligomeric arrangements of the PLH bundles within homomeric ion channels by building models using generic restraints. In particular, the distance between two neighbouring PLHs was bounded both below and above in order to avoid steric clash and allow proper packing. The resulting models provide a theoretical representation of the accessible space for oligomeric arrangements. While the represented space is confined, it encompasses nearly all the ion channel PLH bundles for which the structures are currently known. For a multitude of channels, gating models suggested by paths within the confined accessible space are in qualitative agreement with those established in previous structural and computational studies. Ion channels conduct ions across membranes in response to external stimuli such as change in membrane potential or the binding of ligands, and have diversified molecular architectures [1] tuned by evolution to carry out distinct functions. However, all ion channels have a common structural component: an ion permeation pathway through a transmembrane domain. In theory, any pore, such as those found in some water-soluble enzymes [2] , can be permeable to ions. However, with some exceptions (for example, ClC channels [3] and two-pore domain K + channels [4] , [5] ), most ion permeation pathways are lined by a parallel oligomeric bundle of relatively straight helices, with identical or homologous sequences arranged with (approximate) rotational symmetry [6] ( Fig. 1a ). In this study we explore the conformational space of the pore-lining helix (PLH) bundles in homomeric ion channels. 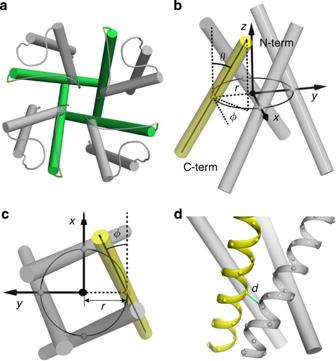Figure 1: Pore-lining helix bundle, modelled as consisting of ideal helices obeying rotational symmetry. (a) Top view of KcsA (Protein Data Bank entry 1BL8), with the pore-lining helix bundle highlighted in green. (b) Side view of an idealized helix bundle. The rotational symmetry axis, pointing towards the N termini of the helices, is defined as thezaxis; the centres of the protomers lie on thexyplane, with theyaxis pointing from the centre of the first protomer (shown in yellow) to thezaxis. The helical axis of the first protomer crosses thexyplane at the point (0, −r, 0) and has polar angleθand azimuthal angleφ. (c) Top view of the idealized bundle. (d) The contact distanced, defined as the closest distance between backbone N, Cα, C and O atoms of two neighbouring helices. Figure 1: Pore-lining helix bundle, modelled as consisting of ideal helices obeying rotational symmetry. ( a ) Top view of KcsA (Protein Data Bank entry 1BL8), with the pore-lining helix bundle highlighted in green. ( b ) Side view of an idealized helix bundle. The rotational symmetry axis, pointing towards the N termini of the helices, is defined as the z axis; the centres of the protomers lie on the xy plane, with the y axis pointing from the centre of the first protomer (shown in yellow) to the z axis. The helical axis of the first protomer crosses the xy plane at the point (0, − r , 0) and has polar angle θ and azimuthal angle φ . ( c ) Top view of the idealized bundle. ( d ) The contact distance d , defined as the closest distance between backbone N, C α , C and O atoms of two neighbouring helices. Full size image Compared with helices in water-soluble proteins, transmembrane helices have significantly enhanced stability and much more closely adhere to ideal geometry, because of their low-dielectric environment and the reduced competition from water and polar side chains for hydrogen bonding with backbone amides and carbonyls [7] . These observations at least partly explain why PLHs in ion channels are relatively straight. In forming a transmembrane domain, helices must be closely packed to provide adequate tertiary and quaternary stability [8] . For PLH bundles, close packing between neighbouring helices is also a functional requirement, since ion permeation necessitates a tightly sealed pore. As shown recently, when large crevices occur between neighbouring PLHs, lipids can enter and occlude the pore [9] . On the other hand, the distance between two neighbouring PLHs cannot be too short; otherwise a steric clash would occur. The fact that PLHs are relatively straight and the distances between adjacent members fall in possibly a narrow range led us to hypothesize that the accessible conformational space for each PLH bundle is rather confined. A confined conformational space would significantly increase the chance of producing similar structures—through convergent evolution—for PLH bundles in unrelated ion channels. Consistent with this idea, two trimeric ligand-gated channels, the zebrafish P2X4 receptor and the chicken acid-sensing ion channel 1a (ASIC1a), have their PLHs arranged in similar conformations even though the two receptors are unrelated in amino-acid sequence and differ in overall structure [10] , [11] . A confined conformational space may also help PLH bundles to preserve their structures as channel proteins undergo exon shuffling and other changes during evolution. For example, two families of tetrameric channels, K + channels and ionotropic glutamate receptors (iGluRs), have similar pore architectures [12] , [13] —as initially postulated based on weak sequence identity for this region [14] , [15] —but share little in sequence and structure elsewhere or in functional characteristics. Channel proteins must cycle through multiple functional states. Correspondingly, PLH bundles must have several stable conformations, at least one with a closed pore and one with an open pore. The paths connecting these conformations constitute a key aspect of channel-gating mechanisms. In addition to the stable conformations, intermediates along the gating paths must fall mostly within the accessible space. If this space is narrow, then there may only be limited possibilities for the modes of gating motion. In support of this scenario, gating motions of PLHs for a variety of channels have all been described in structural and computational studies as iris-like, that is, a change in pore size arising from twist of the PLH bundle. These include (i) trimeric: P2X4 receptor [16] ; (ii) tetrameric: K + (refs 17 , 18 ) and Na + (ref. 19 ) channels and AMPA-subtype iGluR [13] ; (iii) pentameric: mechanosensitive channel of large conductance (MscL) [20] , Gloeobacter violaceus ligand-gated ion channel (GLIC) [21] , and CorA Mg 2+ channel [22] ; and (iv) heptameric: mechanosensitive channel of small conductance (MscS) [23] . The conformational space of transmembrane helix bundles has received previous attention. Sequence analyses have identified prevalence of motifs consisting of small residues (for example, Ala and Gly) in helix–helix packing interfaces as well as certain residue pairs across these interfaces [24] , [25] , [26] , [27] , [28] . Conformational searches, sometimes restrained by such sequence rules and experimental data, were used to build models for particular dimeric and higher oligomeric transmembrane helix bundles [29] , [30] , [31] , [32] . Regarding PLH bundles, based on a model of infinite cylinders arranged with rotational symmetry, Spencer and Rees [6] found a relation between the minimum pore radius and the helix tilt angle. In this study we present a global exploration of the conformational space accessible to PLH bundles and test the hypothesis that this space is very confined. To that end we built structural models of PLH bundles using ideal helices and enforcing rotational symmetry. The tilt angle of each PLH and the contact distance between neighbouring PLHs were limited to ranges observed in helical membrane proteins in the Protein Data Bank (PDB). The latter restraint, on interhelical distance, eliminated most of the starting models (because of either poor packing or steric clash). The surviving models provide a theoretical representation of the accessible region in the full oligomeric arrangement space. This region is indeed confined, but nevertheless contains the PLH bundles of nearly all the homomeric ion channel structures currently described in the PDB. A channel structure outside the putative accessible region may reflect distortion by the membrane mimetic used in structural determination. PLH bundles in the accessible region have four types of gross appearances, with the bundle twist either right-handed or left-handed and the smaller pore opening towards either the N termini or C termini. For each type, expansion in pore size, a signature of channel opening, follows a distinct path, that is, a combination of helix translation and rotation leading to iris-like twist of the PLH bundle. Many gating models developed in previous structural and computational studies follow these calculated paths. Representation of and restraints on PLH bundles To explore the conformational space of PLH bundles in homomeric ion channels, we modelled the helices as ideal, consisting of 24 residues, and assumed rotational symmetry for each bundle ( Fig. 1b–d ). The number, N , of protomers in the PLH bundles ranged from 3 to 7 (with some data also shown for N =8). We defined a coordinate system ( Fig. 1b,c ) with the z axis along the axis of rotational symmetry and pointing towards the N termini of the helices, y axis along the direction from the centre of the first protomer (defined as the centre of geometry of the C α atoms) to the z axis, and x axis along the tangent of the circle containing the centres of all the protomers. If the helix bundle is embedded in a membrane, then the z axis would be along the membrane normal and the xy plane would be parallel to the membrane plane. The oligomeric arrangement of a bundle is fully specified by three coordinates of the first protomer ( Fig. 1b,c ): the radial distance r of its centre and the polar angle θ and azimuthal angle φ of its helical axis (defined as the longest principal axis calculated on the C α atoms and pointing from the C- to the N terminus). Since our model building assumed ideal helices and rotational symmetry, we wanted to verify how well such idealization represents the PLH bundles in actual channel structures. To that end we collected 39 unique channel structures from the PDB (including 4 trimers, 23 tetramers, 9 pentamers, 1 hexamer and 2 heptamers; Supplementary Table 1 ). For each PLH bundle, we produced an idealized substitute, by replacing ideal helices for the protomers and then rotationally symmetrizing the ideal helices. Most of the 39 PLH bundles have relatively small deviations from their idealized substitutes (C α root-mean-square-deviations (RMSDs) <1.5 Å for all but seven bundles; Fig. 2 ), thus justifying our idealization of PLH bundles in the model building. 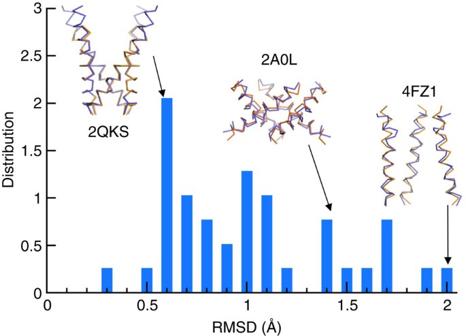Figure 2: Distribution of the CαRMSDs between the pore-lining helix bundles in 39 channel structures and their idealized substitutes. Superposition to idealized substitutes (orange) is shown for Kir3.1 (PDB 2QKS), KvAP (PDB 2A0L) and ASIC1a (PDB 4FZ1) (blue), with low (0.6 Å), medium (1.4 Å), and high (2.0 Å) RMSDs, respectively. Figure 2: Distribution of the C α RMSDs between the pore-lining helix bundles in 39 channel structures and their idealized substitutes. Superposition to idealized substitutes (orange) is shown for Kir3.1 (PDB 2QKS), KvAP (PDB 2A0L) and ASIC1a (PDB 4FZ1) (blue), with low (0.6 Å), medium (1.4 Å), and high (2.0 Å) RMSDs, respectively. Full size image The radial distance r is an important determinant of pore size. A PLH bundle with a very small (or large) r can produce a closed (or open) pore that may take excessive conformational rearrangements in order to reach an open (or closed) state. Therefore, we expected r to fall in some intermediate range. Indeed, nearly all the PLHs in the 39 channel proteins have 5 Å< r <14 Å (calculated on idealized substitutes; Supplementary Table 1 and Supplementary Fig. 1a ). Below we mostly consider models in this range of r ; however, our main conclusions did not change when the upper bound of r was increased to 16 Å. The polar angle θ is commonly referred to as the helix tilt angle. As noted by Bowie [33] and by Spencer and Rees [6] , transmembrane helices tend to be aligned along the membrane normal. Consistent with their observation, the tilt angles of 171 transmembrane helices in 26 proteins [28] are essentially all below 60° ( Supplementary Fig. 1b ). Similarly, the 169 PLHs in the 39 channel proteins have the tilt angles within this range (calculated on idealized substitutes; Supplementary Table 1 and Supplementary Fig. 1c ). Therefore, we focused on models with θ between 0° and 60°; however, increasing the upper bound to 80° did not change our conclusions. As suspected, in order to ensure close packing but avoid steric clash, contact distances (denoted as d , defined as the shortest interhelical distance calculated on backbone atoms; Fig. 1d ) between nearest-neighbour helices in the 26 transmembrane domains fall in a narrow range, from 2.7 to 6.8 Å, peaking ~3.2 Å ( Supplementary Fig. 1d ). Similarly, contact distances of PLHs with neighbouring helices (whether pore-lining or not) are limited to the range of 3.3–6.0 Å, although the peak is now ~5 Å ( Supplementary Fig. 1e ). This upshift in the peak value of d perhaps suggests that PLHs, compared with helices in other transmembrane domains, are somewhat less tightly packed, possibly because of the presence of the pore (a packing ‘defect’). The less tight packing, particularly noted in MscS previously [34] , could facilitate the conformational transitions during channel gating. When contact distances are calculated only between PLHs, the distribution in d expectedly shifts towards higher values, but are still below 7 Å except for 2 of the 39 cases ( Supplementary Fig. 1f ). In our model building we limited the contact distance between PLHs to the 3–7 Å range. Most of our calculations involved only backbone atoms; however, for calculating pore radius we included side chains modelled as alanines. The side chain atoms (as well as backbone atoms of non-nearest neighbouring PLHs when N ⩾ 4) occasionally resulted in steric clash, and such models were also eliminated. The accessible conformational space of PLH bundles is narrow To explore the conformational space of PLH bundles, we built models that uniformly covered the r – θ – φ space with θ in the range of 0°–60°, r in the range of 5–14 Å and φ in its full range (that is, −180° to 180°). The restraint on the interhelical contact distance (that is, 3 Å< d <7 Å) eliminated most of these starting models. As illustrated by the slice at r =9 Å through the oligomeric arrangement space of tetrameric channels ( Fig. 3a ), the elimination is because of either steric clash (that is, d <3 Å) or poor packing (that is, d >7 Å). Steric clash occurs mostly around | φ |=90° along with large θ , whereas poor packing occurs mostly around φ =0° and ±180° along with small θ . Steric clash between C β atoms (as well as backbone atoms of non-nearest neighbouring PLHs) resulted in the additional elimination of a small fraction of models. On the θ – φ plane, the surviving models cluster in narrow strips that form the shape of the letter ‘W’. 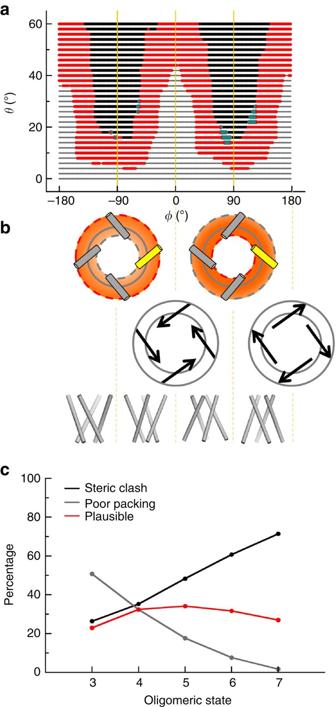Figure 3: Exhaustive exploration of the conformational space accessible to pore-lining helix bundles. (a) A slice (atr=9 Å) through the conformational space for tetrameric bundles. Each starting model is represented by a dot on theθ–φplane. Models that were eliminated byd<3 Å (steric clash), byd>7 Å (poor packing) and by clash between Cβatoms as well as backbone atoms of non-nearest neighbouring helices are coloured in black, grey and teal, respectively; the surviving models are coloured in red. (b) Top row: tilting of the helical axis away from (or towards) thezaxis, corresponding to negative (or positive)φ, results in the larger (or smaller) pore opening towards the N termini located on the red dashed circle. Middle row: bundles with right-handed and left-handed twists have positive and negative cosφ, respectively. Bottom row: helical bundles with four distinct gross appearances, one from each branch of the W-shaped accessible region. (c) Percentages of eliminated (either by steric clash or poor packing) and surviving models in different oligomeric states. Figure 3: Exhaustive exploration of the conformational space accessible to pore-lining helix bundles. ( a ) A slice (at r =9 Å) through the conformational space for tetrameric bundles. Each starting model is represented by a dot on the θ – φ plane. Models that were eliminated by d <3 Å (steric clash), by d >7 Å (poor packing) and by clash between C β atoms as well as backbone atoms of non-nearest neighbouring helices are coloured in black, grey and teal, respectively; the surviving models are coloured in red. ( b ) Top row: tilting of the helical axis away from (or towards) the z axis, corresponding to negative (or positive) φ , results in the larger (or smaller) pore opening towards the N termini located on the red dashed circle. Middle row: bundles with right-handed and left-handed twists have positive and negative cos φ , respectively. Bottom row: helical bundles with four distinct gross appearances, one from each branch of the W-shaped accessible region. ( c ) Percentages of eliminated (either by steric clash or poor packing) and surviving models in different oligomeric states. Full size image Each of the four branches of the W-shaped accessible region spans a 90° range in φ and corresponds to a distinct gross appearance for the PLH bundle, in terms of the orientation of the smaller pore opening (either towards the N termini or C termini) and the handedness of the bundle twist (either right-handed or left-handed). As illustrated in Fig. 3b top row, a bundle with 0°< φ <180° has the N termini closer towards the z axis than the C termini. The opposite is true when –180°< φ <0°. Fig. 3b middle row shows that the bundle twist is right-handed when | φ |<90° and left-handed when 90°<| φ |<180°. The first branch (that is, −180°< φ <−90°) of the W-shaped accessible region thus corresponds to left-handed PLH bundles with smaller openings towards the C termini; and the second (−90°< φ <0°), third (0°< φ <90°) and fourth (90°< φ <180°) branches correspond to right-handed bundles with C-terminal smaller openings and N-terminal smaller openings, and left-handed bundles with N-terminal smaller openings, respectively ( Fig. 3b bottom row). The oligomeric state (that is, N ) was found to affect the proportions of the starting models eliminated because of steric clash and because of poor packing ( Fig. 3c ). Specifically, as N increases, the percentage of models eliminated by steric clash increases, whereas the counterpart by poor packing decreases. This outcome is to be expected, since more protomers in the PLH bundle will bring more chances for steric clash, whereas less protomers will make it more likely to leave gaps between protomers as they are arranged around the circumference of the pore at a given radius. Accounting for model elimination by both steric clash and poor packing and aggregating the results for radial distances in the range of 5–14 Å, pentameric bundles have the highest percentages of surviving models (34.1%; Fig. 3c ), indicating that this oligomeric state has the most freedom in the oligomeric arrangement space. Tetramers, hexamers and heptamers have intermediate percentages of surviving models (32.4%, 31.7% and 27%, respectively), whereas trimers have the lowest percentage of surviving models (23%), implicating an especially confined accessible region. In the r – θ – φ space, the region occupied by the surviving, or ‘plausible’, models is shaped like the letter ‘W’ in three-dimensional (3D) block form (see Fig. 4a,b for tetramers and pentamers and Supplementary Fig. 2a–c for the other oligomeric states). As r increases, poor packing becomes more likely and hence contributes more of the eliminated models. Correspondingly, the top of the W 3D block letter slants towards the θ =60° plane, with reduced thickness. Widening the ranges of r to 16 Å and θ to 80° did not change the confined nature of the accessible region (compare Fig. 4a and Supplementary Fig. 3 for tetramers). For trimers in particular, model elimination because of poor packing accrues to the extent that the second and third (or fourth and first) branches of the W-shaped accessible region are disconnected when r >8.5 Å ( Supplementary Fig. 2a ). 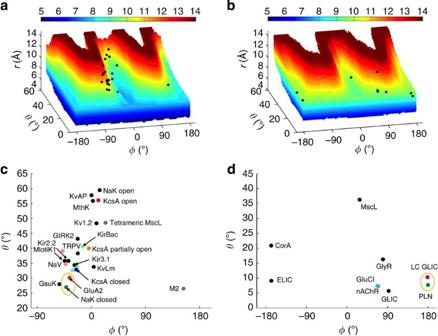Figure 4: The W-shaped accessible region in ther–θ–φspace. (a) The accessible region for tetrameric models, embedding the conformations of 23 actual PLH bundles. Thervalues of the plausible models are displayed according to the colour scale at the top. Each black dot represents an actual PLH bundle. (b) Corresponding results for pentamers. Ina,b, all the black dots are within the respective W shapes (that is, each black dot is within a voxel defined by eight plausible models as vertices that are separated by the smallest increments in (r,θ,φ)). (c,d) The conformations of the actual tetrameric and pentameric PLH bundles displayed on theθ–φplane. In each plot a yellow oval encircles two channels that are either not or only distantly related but have similar conformations for their PLH bundles. Figure 4: The W-shaped accessible region in the r – θ – φ space. ( a ) The accessible region for tetrameric models, embedding the conformations of 23 actual PLH bundles. The r values of the plausible models are displayed according to the colour scale at the top. Each black dot represents an actual PLH bundle. ( b ) Corresponding results for pentamers. In a , b , all the black dots are within the respective W shapes (that is, each black dot is within a voxel defined by eight plausible models as vertices that are separated by the smallest increments in ( r , θ , φ )). ( c , d ) The conformations of the actual tetrameric and pentameric PLH bundles displayed on the θ – φ plane. In each plot a yellow oval encircles two channels that are either not or only distantly related but have similar conformations for their PLH bundles. Full size image Existing structures are mostly found in accessible region To validate the identification of the accessible region of PLH bundles through exhaustive model building, we investigated whether the PLH bundles of the 39 channel structures are actually confined to the putative accessible region. As shown in Fig. 4a,b for the 23 tetramers and 9 pentamers, and Supplementary Fig. 2a–c for the four trimers, one hexamer and 2 heptamers, the oligomeric arrangements of nearly all the PLH bundles in the channel structures fall into the W-shaped accessible region. Besides validating our approach to explore the conformational space of PLH bundles through model building, the fact that the accessible region thus identified fully contains known channel structures provides support for its confined nature. Since the 39 channel structures provided some bounding information for our model building, in theory the outcome that the resulting accessible region fully contains these structures might just reflect the use of this information. However, as described above, the bounds on θ and d are generic features of transmembrane helices, and no restrictions were placed on φ . The only PLH-specific quantity is r but, as we suggested above, its value has to fall in some intermediate range; the precise bounds of r did not seem important since our conclusion remained the same when we went beyond the range found for the 39 channel structures. Even with these bounds, potentially the 39 channel structures could be scattered anywhere in the implicated volume in the r–θ–φ space. Yet they are clustered, and to the same region as identified by our modelling. Two interesting patterns emerge from the display of the PLH bundles in the oligomeric arrangement space. First, the same or related proteins can adopt relatively disparate oligomeric arrangements, although these typically are restricted to the same branch of the W-shaped accessible region. In particular, K + /Na + channels are mostly scattered over the second branch ( Fig. 4c ), pentameric MscL [35] is located on the third branch ( Fig. 4d ), whereas the P2X4 receptor [16] is on the fourth branch in the closed state (PDB 4DW0) but on the first branch in the open state (PDB 4DW1; Supplementary Fig. 2a ). In general, different functional states of the same channel will have disparate oligomeric arrangements, but often not all these states are amenable to structure determination. Second, functionally unrelated channels can adopt very similar oligomeric arrangements. Structural similarities have been noted previously between the P2X4 receptor (PDB 4DW0) and ASIC1a (PDB 3HGC) [10] , [11] ( Fig. 5a and Supplementary Fig. 2a ) and between K + /Na + channels (PDB 2AHY) and iGluRs (PDB 3KG2) [12] , [13] ( Figs 4c and 5b ). Here we identify another case of structural similarity between two unrelated channels: ‘locally closed’ GLIC (LC GLIC; PDB 3TLS) [36] and T-state phospholamban (PLN; PDB 2KYV) [37] ( Figs 4d and 5c ; whether phospholamban is a bona fide Ca 2+ channel is not fully settled [38] , [39] , [40] , [41] ). These structural similarities reinforce the notion that the accessible conformational space of PLH bundles is confined. 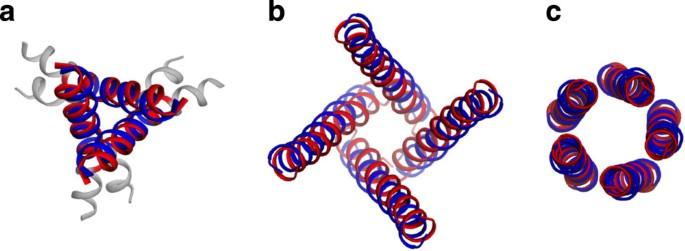Figure 5: Similar conformations for the pore-lining helix bundles of channels that are either not or only distantly related. (a) Superposition of the TM2 helices of desensitized ASIC1a in blue (PDB 3HGC) and apo P2X4 receptor in red (PDB 4DW0). Segments in grey were excluded from superposition. (b) Superposition of the TM2 helices of NaK channel in blue (PDB 2AHY) and TM3 helices of AMPA-subtype iGluR in red (PDB 3KG2), both in the closed state. (c) Superposition of the TM2 helices of locally closed GLIC in blue (PDB 3TLS) and the transmembrane helices of T-state phospholamban in red (PDB 2KYV). Figure 5: Similar conformations for the pore-lining helix bundles of channels that are either not or only distantly related. ( a ) Superposition of the TM2 helices of desensitized ASIC1a in blue (PDB 3HGC) and apo P2X4 receptor in red (PDB 4DW0). Segments in grey were excluded from superposition. ( b ) Superposition of the TM2 helices of NaK channel in blue (PDB 2AHY) and TM3 helices of AMPA-subtype iGluR in red (PDB 3KG2), both in the closed state. ( c ) Superposition of the TM2 helices of locally closed GLIC in blue (PDB 3TLS) and the transmembrane helices of T-state phospholamban in red (PDB 2KYV). Full size image The structure of the open-state P2X4 receptor [16] lies near the border of the accessible region ( Supplementary Fig. 2a ). It is also one of the only two cases where the interhelical distance, at 7.9 Å, exceeds our upper bound of 7 Å ( Supplementary Fig. 1f ), suggesting poor PLH packing. Our molecular dynamics simulations showed that the large crevices between neighbouring PLHs in 4DW1 allow lipids to enter and then occlude the pore [9] . Using a procedure similar to the one here but also incorporating experimental restraints, we generated an open-state model with improved helix packing. The latter is within the accessible region of the oligomeric arrangement space. The second case with excessive interhelical distance is open-state ASIC1a at high pH (PDB 4FZ1) [42] . A d value of 12.1 Å ( Supplementary Fig. 1f ) suggests even worse PLH packing. Correspondingly, this PLH bundle is located well outside the accessible region of the oligomeric arrangement space ( Supplementary Fig. 2a ). Restraint on d leads to distinct distributions of r , θ , φ The shortest interhelical distance d ranges from 3 to 7 Å in channel and non-channel structures. As alluded to above, model elimination because of poor packing (with d >7 Å) and steric clash (with d <3 Å) is uneven as r , θ or φ is varied, leading to characteristic, N -dependent distributions of these coordinates for the plausible models ( Fig. 6 ). 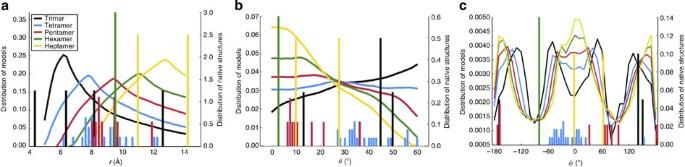Figure 6:N-dependent distributions of ther,θandφcoordinates for the plausible models and for the pore-lining helices of the 39 channel structures. Distributions ofr,θandφare displayed ina–c, respectively. Results are displayed as curves for the plausible models and as bars for the channel structures. Figure 6: N -dependent distributions of the r , θ and φ coordinates for the plausible models and for the pore-lining helices of the 39 channel structures. Distributions of r , θ and φ are displayed in a – c , respectively. Results are displayed as curves for the plausible models and as bars for the channel structures. Full size image As r increases, poor packing contributes more and more while steric clash contributes less and less to model elimination. With increasing N , poor packing overtakes steric clash at successively larger r . Therefore, the r distributions of the plausible models have a maximum, and the maxima move towards larger r at higher N ( Fig. 6a ). Interestingly, the r distributions of the channel structures, despite the relatively small sample sizes, follow the same general N dependence, with r clustered around larger values as N increases. The θ distributions of the plausible models are monotonically increasing for N =3 and 4 but switch to be monotonically decreasing for N =5–7 ( Fig. 6b ). Again, the θ distributions of the channel structures are qualitatively similar. For example, all the trimeric structures but 4FZ1 mentioned above have θ >45°. Similarly, the tetrameric structures have θ values concentrated in the upper half of the range. In contrast, the θ values of the pentameric, hexameric and heptameric structures are mostly restricted to the lower half of the range. The φ distributions of the plausible models have four peaks, around ±45° and ±135°, for N =3 and 4 ( Fig. 6c ). The two inner peaks merge and the two outer peaks shift towards ±180° for N =5–7. The φ values of the channel structures are largely clustered around the peak values of the plausible models. Minimum pore radius depends on all of r , θ , φ Channel opening is generally associated with an increase in the minimum pore radius, R 0 . We calculated the R 0 values for the plausible models and display the results for trimers, tetramers and pentamers in Fig. 7a–c and for higher oligomers in Supplementary Fig. 4 . Models with small R 0 are located at the bottom of the 3D W-shaped accessible region, whereas those with large R 0 are at the top and concentrated around θ =60° and φ =0° or 180°. Potentially, small R 0 and large R 0 locations in the accessible region may represent conformations of closed and open channels, respectively. 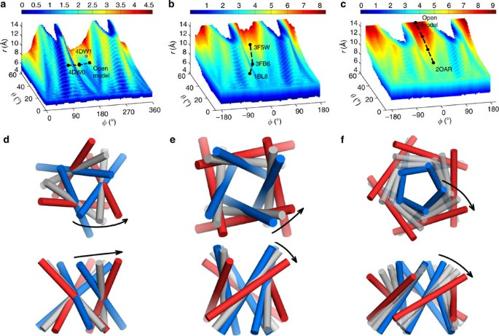Figure 7: Minimum pore radii of the plausible models and gating models of three channels suggested by paths of pore expansion. (a) TheR0values of the plausible trimeric models are displayed according to the colour scale at the top. A path connecting the closed P2X4 receptor (PDB 4DW0) to an open model9represents a hypothetical gating mechanism. The first and second branches are plotted withφshifted by 360° so that the path from the fourth branch to the first branch is connected. The open-state crystal structure (PDB 4DW1) is shown as a grey dot. (b,c) Corresponding results for the tetrameric models and KcsA (path connecting the closed (PDB 1BL8), partially open (PDB 3FB6) and open (PDB 3F5W) states), and for the pentameric models and MscL (path starting from the closed state (PDB 2OAR)), without the shift inφ. (d–f) Illustrations of the gating models for the P2X4 receptor, KcsA and MscL, using conformations shown as black dots ina–c, respectively. Bundles in blue, grey and red represent closed, intermediate and open conformations, respectively, shown in top view (top panels) and side view (bottom panels). Figure 7: Minimum pore radii of the plausible models and gating models of three channels suggested by paths of pore expansion. ( a ) The R 0 values of the plausible trimeric models are displayed according to the colour scale at the top. A path connecting the closed P2X4 receptor (PDB 4DW0) to an open model [9] represents a hypothetical gating mechanism. The first and second branches are plotted with φ shifted by 360° so that the path from the fourth branch to the first branch is connected. The open-state crystal structure (PDB 4DW1) is shown as a grey dot. ( b , c ) Corresponding results for the tetrameric models and KcsA (path connecting the closed (PDB 1BL8), partially open (PDB 3FB6) and open (PDB 3F5W) states), and for the pentameric models and MscL (path starting from the closed state (PDB 2OAR)), without the shift in φ . ( d – f ) Illustrations of the gating models for the P2X4 receptor, KcsA and MscL, using conformations shown as black dots in a – c , respectively. Bundles in blue, grey and red represent closed, intermediate and open conformations, respectively, shown in top view (top panels) and side view (bottom panels). Full size image Clearly, R 0 depends on all the three coordinates r , θ and φ . Overall, R 0 increases as r and θ increase and as φ approaches 0° or 180° (also see Supplementary Fig. 5 ). It is obvious why R 0 increases with increasing r . The increase of R 0 with increasing θ is to some extent an indirect effect. As noted above, with increasing r , close packing of PLHs requires a commensurate increase in θ , as indicated by the slant of the top of the 3D W-shaped accessible region towards the θ =60° plane ( Fig. 4a,b and Supplementary Fig. 2a–c ). Interestingly, the average R 0 value of all the plausible models with a given θ is in reasonable agreement with that predicted by the formula of Spencer and Rees [6] , derived for a model of infinite cylinders (see comparison for pentamers in Supplementary Fig. 5b ). However, for our plausible models, R 0 is not a unique function of θ . Instead, at a given θ , these models show considerable variations in R 0 ( Supplementary Fig. 5b ). R 0 is maximal at φ =0° and 180° because these azimuthal angles correspond to the helical axis of each PLH being tilted tangential to the radial direction. As such the N- and C termini are positioned maximally away from the z axis and hence cannot result in a decrease in pore radius. In contrast, at φ =±90°, the N- and C termini, respectively, are tilted towards the z axis, thereby decreasing the pore radius. Gating models suggested by paths of pore expansion A gating model minimally consists of a path that connects a small R 0 conformation of the PLH bundle to one with an expanded pore size. The confined nature and, in particular, the W shape of the accessible region give rise to limited possibilities for the paths of pore expansion, assuming that intermediates are also mostly confined to the accessible region. As the preceding results on R 0 indicate, such paths generally follow increases in r and θ and approach of φ towards 0° or 180°. These changes in r , θ and φ correspond to helix translations and rotations that have the combined effect of iris-like twists of the PLH bundles, as illustrated below. The P2X4 receptor [16] has r =6.4 Å, θ =49.9° and φ =144.5° in the closed state and r =8.6 Å, θ =45.3° and φ =–159.5° in the open state ( Supplementary Table 1 and Fig. 7a ). Going from the closed (PDB 4DW0) to the open state (PDB 4DW1), while there is little change in θ , r increases significantly (by 2.2 Å) and φ moves significantly (15°) towards 180°, in accord with our expectation. Our remodelled structure for the open state [9] is near 4DW1 but moved inside the accessible region ( Fig. 7a ). The most striking difference between the closed and open states lies in the opposite signs of φ , which place the two states in two different branches of the W-shaped accessible region, corresponding to a switch in the smaller pore opening from facing the extracellular side to facing the intracellular side ( Fig. 7d ). This switch is supported by state-dependent functional data on Ag + accessibility and Cd + coordination [43] . The conformational transition from the closed to the open state may proceed through the ‘bridge’ zone between the fourth and first branches ( Fig. 7a,d ). As noted above, this zone disappears from the accessible region for trimeric channels when r >8.5 Å. Branch crossing is perhaps not expected to be common during channel gating, since it corresponds to substantial conformational changes, akin to those during the functioning of transporters, that involve a switch either in the orientation of the smaller pore opening or in the handedness of the PLH bundle twist. K + /Na + channels span the full range of the second branch ( Fig. 4a,c ). The lower left end, with small θ and near –90° φ , of this branch, along with small r , produces PLH bundles with small minimum pore radii, whereas the upper right end, with large θ and near 0° φ , along with large r , produces PLH bundles with large minimum pore radii. In accordance, K + /Na + channel structures located near the lower left end have been characterized as in the closed state [12] , [13] , [19] , [44] and those near the upper right end have been characterized as in the open state [45] , [46] , [47] , [48] . For a given protein in the K + /Na + channel families, channel opening may follow the path of pore expansion, along the direction from the lower left end to the upper right end. This is indeed the case for the opening of the KcsA channel ( Fig. 7b,e ), with ( r , θ , φ )=(6.8, 32.9°, –25.1°) for the closed state (PDB 1BL8), (7.8, 40.0°, –4.0°) for a partially open state (PDB 3FB6) and (9.8, 56.1°, 11.8°) for the open state (PDB 3F5W; Supplementary Table 1 ) [12] , [48] . The corresponding motion of the PLH bundle is a typical iris-like twist. As shown in Fig. 5b , the PLH bundles of the AMPA-subtype iGluR (PDB 3KG2) [13] and the NaK channel (PDB 2AHY) [44] have very similar structures in the closed state. The structure of the iGluR in the open state is not available but its gating motion has been studied using targeted molecular dynamics simulations [49] . In the resulting activation model, the movement of the PLH bundle agrees with the path of pore expansion specified above, that is, towards the upper right end of the second branch. The same is true of the activation model developed for the NMDA-subtype iGluR [50] . These more sophisticated studies also provide information on how the action of the stimulus (that is, ligand binding) is propagated to the PLH bundles. That critical information is missing in the present study, since the modelling here is limited to the PLH bundles. Only one structure is available for MscL, for the closed state (PDB 2OAR) [35] , but the structure for the open state and the corresponding gating mechanism have been modelled in a number of studies [51] , [52] , [53] , [54] , [55] , [56] . The PDB entry 2OAR has ( r , θ , φ )=(8.4, 36.3°, 28.2°; Supplementary Table 1 and Fig. 7c ). We propose the conformation corresponding to the nearest maximum in R 0 as the open state. This conformation has ( r , θ , φ )=(14.0, 60.0°, 0.0°). The interpolating path between 2OAR and the open model then represents our gating model ( Fig. 7c,f ). The resulting iris-like twist of the PLH bundle is very similar to one proposed by Sukharev et al . [51] , which was validated by crosslinking experiments [20] , [51] and qualitatively recovered in other modelling studies [52] , [55] , [56] . Indeed, our open model agrees well with that of Sukharev et al . [51] ( Supplementary Fig. 6 ), except that the latter has a slightly larger radial distance and larger tilt angle, leading to an even wider pore. We have carried out a global exploration of the conformational space of PLH bundles in homomeric ion channels and found that the accessible region is rather confined. This finding has important implications for the possibilities of channel structures and gating models. PLHs can form proper packing in only a small region of the conformational space. Specifically, the distance between two neighbouring PLHs is delimited by both a lower bound and an upper bound. An overly short distance would lead to steric clash, whereas an overly long distance would lead to poor packing and not produce a tightly sealed membrane-spanning pore. PLHs are typically surrounded by outlying helices, which could further restrict the possible arrangements of the PLH bundles. The confined nature of the accessible conformational space of PLH bundles is reminiscent of the Ramachandran diagram for protein backbone torsion angles, where only a small region is accessible as the other combinations of torsion angles all involve steric clash [57] . The Ramachandran diagram can be viewed as a basis for the fact that there are only two main types of secondary structures, that is, helices and β-strands. The requirement of proper packing of these secondary structure elements is perhaps an explanation for the now commonly accepted assumption that the number of protein tertiary folds is finite [58] , [59] . Our focus here is a quaternary-level structural component that is critical for protein function, that is, the PLH bundle. That the PLH bundles of nearly all the ion channel structures in the PDB are found in the putative accessible region is an important validation of its confined nature. Moreover, cases of proximity in the accessible region have been identified for functionally unrelated ion channels. On the other hand, with the exception of one of the four branches in one oligomeric state, this confined conformational space is still only sparsely populated by current structures. One may ask whether new structures in each oligomeric state will ever fill up the full accessible region to the extent observed now for tetramers in the second branch. We note that the open state of a channel protein is often less amenable to structure determination than the closed state. The confined nature of the accessible conformational space can probably facilitate structure prediction in this context. We have described the oligomeric arrangements of PLH bundles by the three coordinates r , θ and φ . While the radial distance and the tilt angle are commonly used, the azimuthal angle is less so. However, as shown here, this angle on its own defines the gross appearance of the PLH bundle, in terms of the handedness of the bundle twist and the orientation of the smaller pore opening. Correspondingly, the accessible region has a W shape, with four branches for the four types of gross appearance. On the basis of a survey of helical transmembrane domain structures in the PDB, it has been suggested that these structures, because of relatively weak tertiary and quaternary interactions, are potentially sensitive to perturbations by membrane mimetics used in structure determination [8] . The resulting structural distortion could lead to misinterpretation of functional mechanisms. Accordingly, a set of guidelines was proposed for recognizing possible distortion, including poor helix packing and lack of oligomeric symmetry. The accessible conformational space generated here can serve as a practical tool for detecting distortion involving the functionally critical PLH bundles. Among the 39 channel structures analysed here, the open P2X4 receptor (PDB 4DW1) has its PLH bundle located near the border of the accessible region. Potential structural distortion and remodelling of this open state were presented previously [9] . The one case well outside the accessible region, with loose packing between PLHs, is open-state ASIC1a at high pH (PDB 4FZ1). It will require functional studies to validate this structure and provide information for possible remodelling. The confined nature of the accessible conformational space can also facilitate the remodelling of distorted structures. Many gating models have been developed for individual channel proteins in previous studies. Here we took a global view and looked for generic features in gating motions involving PLH bundles. A signature of channel opening is the expansion in pore size. Given the confined nature and especially the W shape of the accessible conformational space, there are limited possible paths of pore expansion for a given channel protein. In a number of cases (for example, KcsA and MscL), the number of such paths narrows down to one and the resulting gating models are qualitatively consistent with those developed in previous structural and computational studies. In other cases (for example, the P2X4 receptor) the channel protein apparently selects one of these possible paths as the gating mechanism. We have assumed that the PLHs are straight and do not bend during gating. Helix bending may generate additional modes of gating motion. The pore size in our modelling here is mostly dictated by the backbone arrangement of the PLHs and essentially free of side chain-specific information. As such this approach will not directly reveal the gating mechanism for cases where the activation gate is formed by bulky side chains. Possible examples of such cases include GLIC [7] , [60] , [61] and MscS [23] . The constriction formed by the bulky side chains may be located away from the minimum pore calculated by our approach and, since the latter does not form the gate, its size in the closed state does not have to become as small as required for preventing ion permeation. Still, the closed state must be located in the accessible region identified by our approach. In addition, for heptamers in particular, a large pore size (potentially representing the open state) can be generated with large r without significant limitation on θ and φ ( Supplementary Fig. 4b ), and hence the choices of gating models are more than those for the lower oligomers. The requirement of proper PLH packing has an impact on lower oligomers differently from higher oligomers. Trimers tend to have small radial distances but large tilt angles, whereas the opposite is true of heptamers ( Fig. 6 ). Correspondingly, trimers tend to produce small minimum pore radii, whereas heptamers tend to produce large ones ( Supplementary Fig. 5 ). The latter result may explain some of the disparities in single-channel conductance between channels of different oligomeric states (10–30 pS for trimers [62] , [63] ; 100–300 pS for tetrameric channels [64] , [65] ; and 1–3 nS for higher oligomers [66] ). Pores formed by even higher oligomeric helix bundles may be always open. Indeed, our octameric models in the accessible region all have pore radii greater than 2.3 Å ( Supplementary Fig. 4c ), which is barely smaller than the radii of hydrated Na + (2.4 Å) and K + (2.7 Å) [67] . To the best of our knowledge, ion channel structures with N >7 do not exist in the current PDB and might not exist at all, possibly because it is difficult for such high oligomeric helix bundles to form a closed state. Therefore, it perhaps is not a coincidence that the most abundant channel structures in the PDB are tetramers and pentamers. The pores in these oligomeric states are neither too small nor too large, allowing for easy access to both the closed and the open states, a hallmark of ion channels. Model generation for PLH bundles For each oligomeric state from trimer to octamer, we generated plausible models by first uniformly sampling the oligomeric arrangement space and then filtering to eliminate those with poor helix packing or steric clash. This two-stage procedure is similar to one used for generating an open-state model for the P2X4 receptor [9] . The coordinate system and the ( r , θ , φ ) coordinates defining the oligomeric arrangement of a PLH bundle are illustrated in Fig. 1b,c . In the sampling stage, we covered r in the range of 5–14 (or 16) Å with an increment of 0.2 Å; θ in the range of 0°–60° (or 80°) with an increment of 2°, and φ in its full range (that is, −180° to 180°) with an increment of 2°, resulting in a total of 256,680 (or 413,280) starting models. The helix rotation angle was not varied. Atomic Cartesian coordinates for these models were generated by running a Tcl script in VMD [68] , with the following steps. ( i ) The first protomer, an ideal α-helix consisting of 24 alanines, was initially placed, with the centre of geometry of the C α atoms at the origin of the coordinate system and the longest principal axis calculated on the C α atoms (pointing from the C- to the N terminus) aligned to the z axis. ( ii ) The first protomer was then moved to its final position in the helix bundle by a sequence of transformations: rotation around the y axis by an angle θ ; rotation around the z axis by an angle φ ; and translation along the y axis by a distance r . ( iv ) Finally, the first protomer was replicated to produce the other protomers by successive rotations around the z axis by 360°/ N . In the filtering stage, the shortest interhelical distance, d , calculated on backbone N, C α , C and O atoms ( Fig. 1d ) between the first and second protomers of each starting model was calculated. Models with d <3 Å were deemed to have steric clash, whereas those with d >7 Å were deemed to have poor helix packing; both were eliminated. In addition, models with a radial distance <1.93 Å for any heavy atom (see below) were deemed to have steric clash and hence also eliminated. The surviving models are referred to as plausible PLH bundles. Calculation of minimum pore radius The minimum pore radius of each plausible PLH bundle was initially calculated using the HOLE programme [69] . As our models contain only PLHs, which do not necessarily seal the pore throughout its length, for a small fraction of the plausible bundles the HOLE programme produced spurious results. We thus sought a robust alternative method for calculating the minimum pore radius, and found that the minimum radial distance of heavy atoms, when offset by 1.93 Å (which is the radius of alanine C β in HOLE), agrees very well with the minimum pore radius calculated by the HOLE programme. All reported minimum pore radii were based on calculating the minimum radial distances. Collection and analysis of ion channel structures We collected a set of 138 ion channel structures from the current PDB, guided by the MPStruct website ( http://blanco.biomol.uci.edu/mpstruc ). Not included were a few structures with incomplete (for example, PDB 3RBZ for the MthK channel) or highly asymmetric (for example, PDB 2QTS, 3S3X, 3S3W and 4FZ0 for ASIC1a) PLHs. PDB entry 2ZW3 (gap-junction channel) was excluded because this channel conducts both ions and small molecules and hence has a much wider pore than typical ion channels. On the other hand, nicotinic acetylcholine receptors were included, whose PLHs are not identical but homologous and obey pseudo fivefold symmetry. A complete list of the channel structures, including the start and end residues of their PLHs, is given in Supplementary Table 1 . When one channel had multiple PDB entries, we retained for later analysis only the ones either putatively representing distinct functional states or otherwise ‘unique’ based on superposition of the PLH bundles. A total of 39 unique structures for 30 different channels were retained ( Supplementary Table 1 ), including 4 trimers, 23 tetramers, 9 pentamers, 1 hexamer and 2 heptamers. Each of the retained structures was assigned an idealized substitute. To that end, the longest principal axis of the PLH bundle (calculated on the C α atoms and pointing from the C- to the N termini) was aligned to the z axis, and each PLH was then superimposed (using C α atoms) to a 24-residue ideal helix. When the PLHs were longer than 24 residues, a 24-residue segment containing the narrowest opening of the bundle was chosen. In rare cases (PDB 4GX5 for GsuK and PDB 3E86 for NaK), the PLHs were significantly bent so a shorter, relatively straight segment was selected for superposition. When the PLHs (or selected segments thereof) were shorter than 24 residues, the number of superimposed C α atoms was less than 24. In all cases, the same segment was used for the superposition of all the protomers in a given PLH bundle; these segments are listed in Supplementary Table 1 . The idealized substitute of the PLH bundle was obtained by symmetrizing the ideal helices superimposed to the individual PLHs. Specifically, the ( r , θ , φ ) coordinates as well as the helix rotation angle of each ideal helix were calculated (using all the 24 C α atoms). The average of each coordinate was then taken over the protomers. These average coordinates were then used to generate the idealized substitute, by running the same Tcl script described above, except with the additional move in step ( i ) that the helix was rotated around its axis to the desired helix rotation angle. The C α RMSDs of the PLH bundles in the channel structures from their idealized substitutes, calculated over the segments listed in Supplementary Table 1 , are reported in Supplementary Table 1 and Fig. 2 . To make direct comparison with the models that we generated from uniform sampling, we used the ( r , θ , φ ) coordinates calculated on the idealized substitutes ( Supplementary Table 1 , Figs 4 , 6 and 7 , and Supplementary Figs 1 and 2 ). Similar calculations were made on a set of 26 transmembrane proteins collected previously [28] ; all but seven of the latter proteins were not ion channels. How to cite this article: Dai, J. and Zhou, H.-X. General rules for the arrangements and gating motions of pore-lining helices in homomeric ion channels. Nat. Commun. 5:4641 doi: 10.1038/ncomms5641 (2014).